A new Late Triasssic phytogeographical scenario in westernmost Gondwana Floral provincialism within the Southern Hemisphere during the Late Triassic (230 Ma) is characterized by the Ipswich and Onslow provinces, recognized originally in eastern Gondwana. However, new palynological assemblages from the Ischigualasto Formation, northwestern Argentina (231–225 Ma), change the phytogeographic interpretation for the Carnian–Norian in the westernmost Gondwana, which was previously considered part of the southern floral Ipswich province. Here we show the presence of diagnostic Euramerican species within assemblages dominated by Gondwanan taxa that allows us to refer the palynofloras to the Onslow province. Our new data extend the Onslow floral belt, previously recognized from the western edge of Tethys to Timor, to the western margin of South America. This has implications for palaeophytogeography, palaeoclimate reconstructions and the palaeoecology of a Triassic ecosystem, which has yielded significant vertebrate remains and is regarded important in the early evolution of groups such as the Dinosauria. All continents coalesced to form the supercontinent Pangaea during the Triassic. However, the supercontinent began to divide in the Middle Triassic into Laurasia and Gondwana, separated by the roughly equatorial Tethys ocean ( Fig. 1 ). The Dicroidium flora characterizes the Triassic of Gondwana and constitutes a phytogeographic realm [1] , [2] , [3] . Two palynological phytogeographic areas are recognized within Gondwana for the Middle–Late Triassic: the Ipswich and the Onslow provinces, which coincide with latitudinally constrained vegetation floral belts [2] , [3] , [4] . The Onslow province represents a mixture of Gondwanan and European taxa recognized in northwestern Australia, northwest Madagascar, East Africa, Indian Godavari, South Rewa and Manahadi basins, and connected East Antarctic Lambert Graben. The Ipswich province developed in southern and eastern Australia, Transantarctic Mountains region, South Africa and Argentina, with typical Gondwanan species ( Fig. 1a ). The Ipswich palynofloras represent cool temperate plant communities and the Onslow palynoflora reflects vegetation of warm temperate climates as it contains elements from the equatorial Tethyan phytogeographic realm. 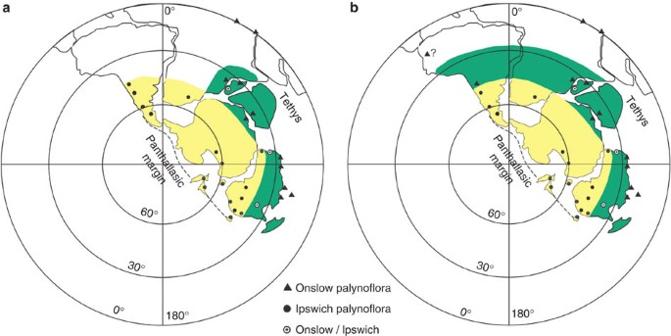Figure 1: Gondwanan distribution of Onslow and Ipswich microfloras. (a) Distribution of Ipswich and Onslow palynofloras suggested by previous authors5,7. (b) Phytogeography proposed in this paper, based on the new data from Ischigualastian palynofloras. Note that data from the circum-Mediterranean area are in the Northern Hemisphere. Figure 1: Gondwanan distribution of Onslow and Ipswich microfloras. ( a ) Distribution of Ipswich and Onslow palynofloras suggested by previous authors [5] , [7] . ( b ) Phytogeography proposed in this paper, based on the new data from Ischigualastian palynofloras. Note that data from the circum-Mediterranean area are in the Northern Hemisphere. Full size image The European taxa of the Onslow palynofloras mainly include the genera: Aulisporites , Camerosporites, Enzonalasporites , Infernopollenites, Minutosaccus, Ovalipollis and Samaropollenites , all of which are absent from the Ipswich palynofloras [4] , [5] , [6] , [7] . Carnian miospore assemblages extending from the western edge of Tethys to its southeastern shorelines, for example, Timor, have been included in the Onslow province [6] . The occurrence in the Northern Hemisphere of the index species Samaropollenites speciosus , and other typical southern elements of Onslow palynological affinity, supports the existence of a homogeneous parent plant community that grew under the influence of an equable, warm and humid climatic regime controlled by monsoonal circulation [7] . However, these Circum-Mediterranean assemblages were also considered as ‘mixed’ [5] but still distinct from the Onslow-type palynofloras. The Triassic palynological record of South America is scarce and mainly concentrated in Argentina [8] . Within the country, this record extends from the Lower Triassic to the Upper Triassic, including the assemblages from the Cacheuta, Cerro Puntudo, Chihuido, Comallo, El Tranquilo, Las Cabras, Los Rastros, Paso Flores, Potrerillos, Puesto Viejo, Santa Clara and Rancho de Lata formations (see refs in 9, 10 [9] , [10] ). All these palynofloras have been referred to the Ipswich province although, in many cases, based on few productive samples ( Fig. 1a ). In northwestern Argentina, the Ischigualasto-Villa Unión Basin ( Fig. 2a ) is one of a series of extensional basins developed on the western margin of Pangea during the early Mesozoic [11] . This basin preserves a complete and continuous fossiliferous succession of continental Triassic rocks ( Fig. 2 ). The most notable fossil assemblages are preserved in the Upper Triassic units, especially in the Carnian–Norian Ischigualasto Formation [12] , [13] where tectosedimentary and palaeoclimatic conditions were optimal for vertebrate and plant preservation. The Ischigualasto Formation, located at 40°S palaeolatitude, comprises fluvial sandstones, mudstones and palaeosols deposited during the last stage of synrift tectonics [11] , [14] . Extremely seasonal conditions, arid to semi-arid palaeoclimates are recorded in the sedimentology, taphonomy, ichnology and palaeosols of the lower two members (La Peña and Cancha de Bochas, Fig. 2b ). Semi-humid conditions are reflected in the third member (Valle de la Luna) and a return to semi-arid palaeoclimates is expressed at the top of the formation and the transition to the overlying Los Colorados Formation [11] , [15] , [16] , [17] , [18] . These conditions prevailed during the Late Triassic, a time during which earliest-known dinosaurs [13] , [19] together with archosauromorphs, crurotarsal archosaurs, therapsids and amphibians lived in southwest Gondwana. Furthermore, active channel, abandoned channel and swamp deposits of the Valle de la Luna Member host enormous quantities of mummified leaf cuticles and palynomorphs. However, the Ischigualasto Formation palynological record has not been studied in detail with only two short communications published [20] , [21] . One sample studied from the basal section was grouped with samples from other stratigraphic units in the so called ‘M1’ association, without a precise list of the species identified [20] . Later, two samples from the middle portion of the Ischigualasto Formation were analysed, and based on the presence of abundant Gondwanan genera, an age no older than Norian was proposed for the fossiliferous strata [21] . 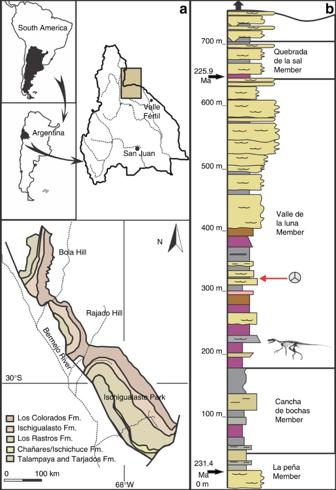Figure 2: Geological setting. (a) Location map and geological map of the Ischigualasto area. (b) Simplified log of the Ischigualasto Formation showing the stratigraphic positions of the studied palynological samples, the first dinosaur findings and radiometric dates. Figure 2: Geological setting. ( a ) Location map and geological map of the Ischigualasto area. ( b ) Simplified log of the Ischigualasto Formation showing the stratigraphic positions of the studied palynological samples, the first dinosaur findings and radiometric dates. Full size image Given the importance of these deposits in terms of early Mesozoic tetrapod evolution and the establishment of typically Mesozoic terrestrial ecosystems, further detail on the plant communities present is invaluable to the study of these Triassic landscapes. We analysed twenty-three palynological samples from a swamp deposit of the Valle de la Luna Member. All the samples contain diagnostic Carnian–Norian species previously recorded in Euramerica and Eastern Gondwana. We applied multivariate analysis to compare our assemblages with other described in those regions, and the results confirm the close relation with the Onslow province. Our analysis also reveals a wider geographic distribution of some Euramerican species during the Carnian–Norian than the previously suspected. Composition of the palynological assemblages The identified palynological assemblages are rather uniform and contain abundant taxa previously recognized elsewhere in Gondwana. All samples are characterized by an abundance (40–85%) of non-taeniate bisaccate pollen including Alisporites australis de Jersey and Falcisporites nuthallensis Balme. Taeniate pollen is abundant (up to 30%) in some samples, and simple monosulcate pollen referred to Cycadopites is also common. Moreover, spores such as Cadargasporites reticulatus de Jersey and Paten ( Fig. 3g ), C. baculatus (de Jersey and Paten) Reiser and Williams, Dictyophyllidites mortoni (de Jersey) Playford and Dettmann, Striatella seebergensis Mädler ( =Duplexisporites problematicus ) ( Fig. 3b ), Playfordiaspora cancellosa (Playford and Dettmann) Maheshwari and Banerji, Rogalskaisporites cicatricosus Rogalska 1954 ex Danze-Corsin and Laveine ( Fig. 3q ), Partitisporites spp. ( Fig. 3h ) among others, usually occur in variable proportions (5–40%). However, the most significant discovery is the occurrence in all the samples of northern or Tethyan species never recorded previously in Argentina: Patinasporites densus Leschik ( Fig. 3e ), Enzonalasporites vigens Leschik ( Fig. 3c ), Vallasporites ignacii Leschik ( Fig. 3d ), Minutosaccus crenulatus Dolby ( Fig. 3k ), Ellipsovelatisporites plicatus Klaus ( Fig. 3l ), Ovalipollis pseudoalatus (Thiergart) Schuurman ( Fig. 3p ), Ovalipollis ovalis Krutzsch ( Fig. 3u ), Triadispora plicata Klaus ( Fig. 3r ) together with typical Onslow-type components such as Samaropollenites speciosus Goubin ( Fig. 3f ), Rimaesporites aquilonalis Goubin ( Fig. 3s ), Polypodiisporites mutabilis Balme ( Fig. 3n ) and Cycadopites stonei Helby ( Fig. 3m ). Four diagnostic species of the Onslow flora [4] are absent in the palynological assemblages, here analysed from the Ischigualasto Formation: Aulisporites astigmosus (Leschik) Klaus , Camerosporites secatus Leschik and Infernopollenites claustratus Dolby and Balme, and Staurosaccites quadrifidus Dolby. However, the latter two species are characteristic of the S. quadrifidus Biozone, which age slightly older than the Ischigualastian [4] , [22] , and A. astigmosus is considered to be facies controlled [5] . 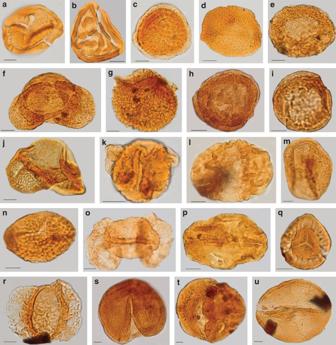Figure 3: Selected representative species of the palynological assemblages from the Ischigualasto Formation. (a)Limatulasporites fossulatus/limatuluscomplex; (b)Striatella seebergensisMädler; (c)Enzonalasporites vigensLeschik; (d)Vallasporites ignaciiLeschik; (e)Patinatisporites densusLeschik; (f,j)Samaropollenites speciosusGoubin; (g)Cadargasporites reticulatusde Jersey and Paten; (h,i)Partitisporitesspp.; (k)Minutosaccatus crenulatusDolby; (l)Ellipsovelatisporites plicatusKlaus; (m)Cycadopites stoneiHelby; (n)Polypodiisporites mutabilisBalme; (o)Chordasporites singulichordaKlaus; (p)Ovalipollis pseudoalatus(Thiergart) Schuurman; (q)Rogalskaisporites cicatricosusRogalska 1954 ex Danze-Corsin and Laveine; (r)Triadispora plicataKlaus; (s,t)Rimaesporites aquilonalisGoubin; (u)Ovalipollis ovalisKrutzsch. Scale=10 μm. Figure 3: Selected representative species of the palynological assemblages from the Ischigualasto Formation. ( a ) Limatulasporites fossulatus/limatulus complex; ( b ) Striatella seebergensis Mädler; ( c ) Enzonalasporites vigens Leschik; ( d ) Vallasporites ignacii Leschik; ( e ) Patinatisporites densus Leschik; ( f , j ) Samaropollenites speciosus Goubin; ( g ) Cadargasporites reticulatus de Jersey and Paten; ( h , i ) Partitisporites spp. ; ( k ) Minutosaccatus crenulatus Dolby; ( l ) Ellipsovelatisporites plicatus Klaus; ( m ) Cycadopites stonei Helby; ( n ) Polypodiisporites mutabilis Balme; ( o ) Chordasporites singulichorda Klaus; ( p ) Ovalipollis pseudoalatus (Thiergart) Schuurman; ( q ) Rogalskaisporites cicatricosus Rogalska 1954 ex Danze-Corsin and Laveine; ( r ) Triadispora plicata Klaus; ( s , t ) Rimaesporites aquilonalis Goubin; ( u ) Ovalipollis ovalis Krutzsch. Scale=10 μm. Full size image Bisaccate pollen dominate the assemblages from the Valle de la Luna Member and many of the diagnostic species are present in low number, as occurs in northern Australia [23] . They may not be detected when are analysed few samples or those with low diversity [23] . Age A late Carnian–early Norian age may be discerned from the presence of the Enzonalasporites–Patinasporites–Pseudoenzonalasporites–Vallasporites group [24] and Samaropollenites speciosus Goubin, Ellipsovelatisporites plicatus Klaus, Chordasporites singulichorda Klaus ( Fig. 3o ), Limatulasporites fossulatus/limatulus complex ( Fig. 3a ) and Ovalipollis pseudoalatus (Thiergart) Schuurman ( Fig. 3p ), some of which seem to disappear in the late Norian of the Northern Hemisphere. Moreover, Cadargasporites reticulatus and C. baculatus are indicative of a Carnian–Norian age in Gondwana [22] . Multivariate analysis Using a combination of cluster analysis and detrended correspondence analysis (DCA), the distribution of selected late Carnian–early Norian diagnostic species has revealed three distinct associations. This analysis was based on published records from Australia (Onslow and Ipswich associations), East India, East Africa, Europe, Circum-Mediterranean area, Timor, United States and the data presented here. Cluster analysis resolves three main groups ( Fig. 4a ). The Onslow, East African, East Indian and Ischigualastian palynofloras constitute a distinctive group. Although sharing species, there is a clear divide between them and the Euramerican assemblages represented by a tightly defined group that essentially corresponds to the Circum-Mediterranean area, Europe and United States. Timor appears to group closest to Euramerican, although it was located in the Southern Hemisphere. Ipswich province is clearly differentiated from the other two clusters. This subdivision is also identifiable on the first axis assemblage’s scores in the DCA and corresponds quite well with what it is known about the distribution of the palynofloras: southernmost assemblages on the left and northern assemblages on the right ( Fig. 4b ). This suggests that the species distribution follows a latitudinal gradient north to south. The position of the East Africa is equivocal: in the cluster analysis it clearly belongs to the Onslow province, but the low axis 1 score on the DCA suggests Euramerican affinities, but this may be just a function of its very-low known species diversity. 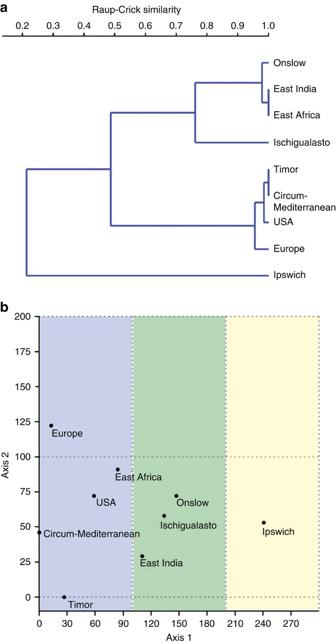Figure 4: Multivariate analysis of selected late Carnian–early Norian species. Species from Australia (Ipswich and Onslow floras), Europe, Circum-Mediterranean area, East Africa, East India, Timor, United States and Ischigualasto Formation. (a) Cluster analysis of Raup–Crick similarity coefficients. (b) DCA of the data for the first two axes (representing 38.3% and 17.1%, respectively, of the variation in the data matrix). Figure 4: Multivariate analysis of selected late Carnian–early Norian species. Species from Australia (Ipswich and Onslow floras), Europe, Circum-Mediterranean area, East Africa, East India, Timor, United States and Ischigualasto Formation. ( a ) Cluster analysis of Raup–Crick similarity coefficients. ( b ) DCA of the data for the first two axes (representing 38.3% and 17.1%, respectively, of the variation in the data matrix). Full size image The palynological analysis of the Valle de la Luna Member (231.4–225.9 Ma) [12] , [13] reveals the first record of diagnostic Tethyan species in southwestern Gondwana and the first conclusive record of an Onslow palynoflora in South America. Although a sparse assemblage composed of Enzonalasporites densus, Minutosaccus sp. cf. M. crenulatus and Samaropollenites speciosus was described from higher latitude in Peru, it is uncertain if it represents a typical Onslow palynoflora [25] . However, the Ischigualastian assemblages are the first described where Cadargasporites specimens are mixed with Onslow or northern species. Mixing assemblages of this Gondwanan species with northern elements have already been reported in Australia [22] and India [33] . Previous data constrain the westernmost extent of the Onslow flora terminated in eastern Africa [26] , with western Gondwana being dominated by Ipswich-type palynofloras. Some of the identified species from the Ischigualasto Formation are important phytogeographic indicators that extend the geographic distribution of the Onslow province to the westernmost Gondwana. This changes substantially the traditional phytogeographic scheme for the Late Triassic proposed originally [4] . Although factors controlling the phytogeography were complex [5] , [22] , the palaeogeographical position of the Ischigualastian palynofloras are consistent with their inclusion in the zone of the Onslow palynofloras ranging from 30 to 40° S ( Fig. 1b ), indicating these vegetational communities were much more widespread than previously thought. In the same way, it has been suggested that the Upper Triassic global palaeogeography supports the similarity between the Circum-Mediterranean and Onslow palynofloras [6] . The analysis of the palynological assemblages described for the Carnian–Norian suggests a widespread distribution of the Enzonalasporites complex, Camerosporites , Rimaesporites -like, Samaropollenites and Ovalipollis pollen together some diagnostic spores. These taxa reach a latitudinal belt spanning the 30–40° to the south where they are mixed with endemic Gondwanan species. Their presence or abundance is probably the result of diverse factors [5] . Taking into account that Ischigualastian depositional settings were similar to those recorded in the eastern Australian basins (Ipswich province), which were dominated by continental sedimentation, the dispersal of these floras seem to be controlled by more local environmental conditions. The apparent constraint during the Carnian–Norian of ‘pure’ Gondwanan assemblages in the southernmost areas ( Fig. 1b ) must be confirmed by more extensive geographic sampling of, and improved age constraints on, Southern Hemisphere Late Triassic palynofloras, analysing more samples by stratigraphic sections, making special emphasis in the chronostratigraphy of the considered areas, because the Triassic interval is poorly constrained because of a scarcity of radiometric ages. The Upper Triassic deposits of the Ischigualasto-Villa Unión Basin reveal a wealth and diversity of well-preserved vertebrate and plant fossils. The plant community (23 species) was dominated by Corystospermaceae [9] and was interpreted as a subtropical riparian sclerophyll forest accompanied by herbaceous-shrubby understory [27] . This was undoubtedly an important evolutionary hotbed that facilitated the speciation of new and novel forms of archosaur (that is, all dinosaur linages), the extinction of others (that is, the archosauromorph Scaphonix ), and the preservation of many species of palaeovertebrates together with an outstanding macroflora, consisting of cuticles, tree trunks and roots [13] , [16] . The enhanced potential for organic preservation in the Ischigualasto Formation (Valle de la Luna Member) was coincident with an increase in humidity, evidenced by changes in the palaeosols, fluvial architecture, in the palaeovertebrate preservation and the appearance of the entire range of palaeofloristic remains, and the quality and abundance of animal and plant remains compared with underlying units [13] , [15] , [16] . This local change appears to coincide with a humid climatic pulse recognized extensively around the Tethys and in southwestern North America during the Carnian as a consequence of the extreme continental monsoonal regime fostered by the Pangean supercontinent [28] , [29] , [30] . Palynological samples We analysed 23 samples of mudstones from a 300-m-long, 8-m-thick swamp deposit ( Fig. 2 ). The sample rocks were given the standard palynological processing treatment: after cleaning and drying, hydrochloric acid and hydrofluoric acid were added to remove the carbonate and silicate minerals respectively. No oxidizing agent was used. The organic residue was sieved and washed thoroughly through a 20-μm nylon sieve. Five slides of each sample were mounted with glycerine jelly. Statistical analysis Cluster analysis and DCA were used in this study. These were all performed using the PAST software Package [31] . We use the Raup–Crick coefficient, which is calculated using a ‘Monte-Carlo’ randomization procedure to determine how often a comparable level of similarity occurs in 200 randomly replicated samples of the same size [32] . Forty-five late Carnian–early Norian diagnostic morphospecies were selected [5] , [6] , [7] , [22] , and their presence–absence in northwestern and eastern Australia (Onslow and Ipswich), East Africa [26] , East India [33] , [34] , Circum-Mediterranean area, Europe, United States and Timor [35] was checked ( Supplementary Table S1 ). Some species have been grouped, such as Alisporites/Falcisporites and Limatulasporites fossulatus/limatulus complex. They show a wide variability and intergradation, and their phytogeographic or full-scale biostratigraphic value is not focused on the presence of a particular species. Some original taxonomic assignments [4] have been preserved for the Onslow palynoflora (for example, Rimaesporites including similar Brachysaccus and Vesicaspora forms). Thus, it promoted a more easy comparison with the original characterization of the Onslow flora. Repository All the palynological slides are housed at the Palynological Collection of the Museo Argentino de Ciencias Naturales ‘B. Rivadavia’ (registered numbers BAPl 6404–6426). How to cite this article: Césari, S. N. et al. A new Late Triasssic phytogeographical scenario in westernmost Gondwana. Nat. Commun. 4:1889 doi: 10.1038/ncomms2917 (2013).